Accelerated single photon emission from dye molecule-driven nanoantennas assembled on DNA A photon interacts efficiently with an atom when its frequency corresponds exactly to the energy between two eigenstates. But at the nanoscale, homogeneous and inhomogeneous broadenings strongly hinder the ability of solid-state systems to absorb, scatter or emit light. By compensating the impedance mismatch between visible wavelengths and nanometre-sized objects, optical antennas can enhance light–matter interactions over a broad frequency range. Here we use a DNA template to introduce a single dye molecule in gold particle dimers that act as antennas for light with spontaneous emission rates enhanced by up to two orders of magnitude and single photon emission statistics. Quantitative agreement between measured rate enhancements and theoretical calculations indicate a nanometre control over the emitter-particle position while 10 billion copies of the target geometry are synthesized in parallel. Optical antennas can thus tune efficiently the photo-physical properties of nano-objects by precisely engineering their electromagnetic environment. Optical antennas are an attractive alternative to microcavities for the broadband enhancement of spontaneous decay rates from solid-state emitters at room temperature [1] , [2] : the width of their resonances is similar to luminescence spectra but the associated low quality factors are compensated by sub-wavelength field confinement. However, as noble metals are lossy, non-radiative decay channels dominate at short emitter–antenna distances due to coupling with multipolar modes [3] . These modes do not radiate efficiently and are described as dark, while the dipolar resonances of nanoantennas are bright as they couple readily to the far-field. Because of overlapping dipolar and multipolar resonances and weak field confinement, spherical silver or gold particles are not efficient antennas [4] but they can be controllably coupled to single molecules (SMs) using atomic force microscopy [5] , [6] . Elongated particles and particle pairs with nanometre gaps have been proposed as more efficient antennas because they offer larger confinements and a bright longitudinal mode red-shifted with respect to lossy high-energy modes [4] , [7] . Reproducible and large-scale interfacing of single emitters with anisotropic nanoantennas is challenging as electromagnetic coupling varies at the nanometre scale with drastic modifications of the local density of optical states [3] , [5] , [6] and of the radiation pattern [8] , [9] . Efficient interaction between a molecule and a nanoantenna was only observed by randomly depositing SMs on e-beam-fabricated bow-tie antennas [10] . Lithography was used to position quantum dots next to gold Yagi-Uda antennas [11] or diamond colour centres in silver nano-apertures [12] ; but the position uncertainty of the emitting transition dipole is several tens of nanometres. On the other hand, synthetic DNA can place SMs in the vicinity of 15-nm-diameter gold nanoparticles (AuNPs) with nanometre resolution [13] but the gold spheres quench spontaneous emission because of negligible scattering cross-sections. To enhance fluorescence instead of suppressing it, nanoantennas require several larger electromagnetically-coupled spheres with interparticle gaps smaller than the AuNP radii [7] . We recently synthesized dimers of 36-nm-diameter AuNPs linked by a single DNA double strand as short as 10 nm, which feature substantial scattering cross-sections [14] . The DNA spacer is stretched by electrostatic interactions in buffer solutions [14] and its length can be changed to tune the distance between the particles and a molecule in the centre of the double strand. In this work, we introduce a single dye molecule on one DNA base and measure enhanced fluorescence decay rates with single photon emission statistics in AuNP dimers. Mie theory calculations indicate that the emitter position is controlled at the nanometre scale. Furthermore, by analysing the antenna behaviours of single AuNPs and dimers, we observe that Purcell factors larger than 100 can be obtained in dimers with increased fluorescence count rates compared with isolated fluorescent molecules, while single AuNPs typically quench spontaneous emission. DNA-driven nanoparticle assembly The interaction between a dye molecule and a particle dimer linked by DNA was already discussed in the literature but inhomogeneous samples prevented a statistical analysis [15] or required atomic force microscopy to correlate nanostructure geometry and Raman scattering properties [16] . To obtain homogeneous samples of SM-featuring AuNP dimers, we use electrophoresis to purify gold particles conjugated preferentially to one DNA strand [17] and, after hybridization of complementary sequences, AuNP dimers linked by a single double strand [18] . In this study, we employ two 30 bases and 50 bases DNA sequences with a single ATTO647N molecule in the centre (respectively attached to amino-modified C and A bases, making this fabrication technique compatible with most water-soluble organic dyes). Both strands feature a trithiolated moiety at the 5′ end that binds covalently to the AuNPs without being removed when the gold surface is passivated with thiolated ethylene glycol oligomers (PEG) [19] . Using the procedures and DNA sequences described elsewhere [14] , we purify 36-nm-diameter PEG-stabilized AuNPs linked to one DNA single strand that are then hybridized in dimers. Dimer suspensions exhibit purities of 70% and interparticle distances of 13±1 nm and 17.5±1.5 nm, respectively, for 30 base pairs (bp) and 50 bp spacers as estimated in cryogenic electron microscopy (cryo-EM) [14] . The PEG shell of the particle that carries the ATTO647N molecule is methyl terminated while the surface of the AuNPs linked to the complementary strand features biotin molecules. Biotin binds to the neutravidin-functionalized walls of microfluidic chambers used for single-molecule fluorescence experiments [14] , [19] . By adding biotin to the AuNP that does not carry a dye molecule, we ensure that, in dimer samples, leftover single particles with an ATTO647N will not bind to the chamber. To couple ATTO647N molecules to a single gold particle, we hybridize SM-conjugated AuNPs to a complementary strand exhibiting a biotin moiety at the 5′ end. Free dye-modified DNA strands are also hybridized to the biotin-modified strand to compare the fluorescence properties of SMs in three geometries as depicted in Fig. 1a : isolated, linked to one AuNP and in the centre of a dimer. A typical cryo-EM image of 30 bp dimers is given in Fig. 1b . Suspensions of dimers and mono-conjugated AuNPs are prepared for both DNA linker lengths in 20–50 fmole quantities. 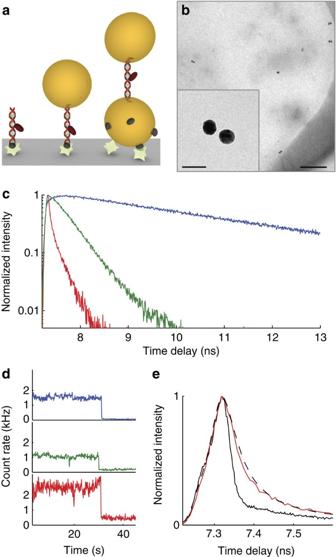Figure 1: SM fluorescence lifetimes and time traces. (a) Representation of the three studied samples bound to a glass cover slip (black dots correspond to biotin and grey prisms to NeutrAvidin). In practice, the 36-nm particle diameter is three times larger than the length of the DNA spacer. (b) Low and high (inset) magnification Cryo-EM images of the 30-bp dimer sample (scale bars =500 and 50 nm, respectively). (c) Typical fluorescence lifetimes and (d) corresponding time traces (100 ms averaging) of ATTO647N molecules for an isolated emitter (blue solid line, 3200±150 ps lifetime), a single AuNP with 50 bp spacer (green solid line, 310±10 ps lifetime) and a 30 bp dimer (red solid line, 35±5 ps lifetime). (e) IRF (black solid line) convoluted with a single exponential decay (black dashed line) used to fit the lifetime (35±5 ps) of the molecule on a 30 bp dimer (red line). Figure 1: SM fluorescence lifetimes and time traces. ( a ) Representation of the three studied samples bound to a glass cover slip (black dots correspond to biotin and grey prisms to NeutrAvidin). In practice, the 36-nm particle diameter is three times larger than the length of the DNA spacer. ( b ) Low and high (inset) magnification Cryo-EM images of the 30-bp dimer sample (scale bars =500 and 50 nm, respectively). ( c ) Typical fluorescence lifetimes and ( d ) corresponding time traces (100 ms averaging) of ATTO647N molecules for an isolated emitter (blue solid line, 3200±150 ps lifetime), a single AuNP with 50 bp spacer (green solid line, 310±10 ps lifetime) and a 30 bp dimer (red solid line, 35±5 ps lifetime). ( e ) IRF (black solid line) convoluted with a single exponential decay (black dashed line) used to fit the lifetime (35±5 ps) of the molecule on a 30 bp dimer (red line). Full size image Single-molecule fluorescence lifetime measurements To minimize photobleaching and blinking of SMs, we add an oxygen scavenger [20] and reducing and oxidizing agents [21] , [22] in the microchamber. The sample is illuminated with a pulsed supercontinuum source spectrally filtered at 635 nm. Weak excitation intensity of 200 W cm −2 ensures that the fluorescence experiments are performed without SM saturation. The fluorescence signal, at 670±25 nm, is imaged on an EMCCD camera to ensure that it corresponds to a diffraction-limited spot, or focused on an avalanche photodiode (APD) after confocal spatial filtering. Time-correlated single photon counting is used to estimate the fluorescence lifetime of SMs with a 75±5 ps full-width at half maximum of the instrument response function (IRF). Fluorescence lifetimes and time traces for the three sample geometries are given in Fig. 1c and d (a photobleaching step confirms the emitter singularity). To estimate the emission rate, we convolute the IRF with a monoexponential decay and fit the fluorescence data [10] as shown in Fig. 1e for an ATTO647N molecule in a 30 bp dimer. In this case, the lifetime is 35±5 ps, 91 times shorter than the isolated dye of Fig. 1c (3,200 ± 150 ps). We performed 420 lifetime measurements on diffraction-limited spots from isolated ATTO647N molecules, single AuNPs and dimers for both 30 bp and 50 bp spacers. From these measurements, 81% could be fitted with the IRF convoluted with a single exponential decay while 8% featured weak signal to noise ratios (owing to early photobleaching) and 11% biexponential decays (owing to a large background signal or more than one molecule in the focal volume). Single lifetimes and stable fluorescence time traces indicate that the SM orientations are stable during the measurement. Complete rotational hindrance of similar cationic dye molecules bound to double-stranded DNA was recently analysed in time-resolved anisotropy measurements [23] . 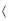Figure 2: Distributions of decay rate enhancementsΓ/Γ0. Isolated ATTO647N molecules (a), single AuNPs with 50 bp (b) and 30 bp (c) DNA spacers, and 50 bp (d) and 30 bp (e) dimers. Experimental bar widths are ΔΓ/Γ=Δτ/τ=0.12. The solid black line in (a) is a Gaussian fit of the experimentalΓ0/Γ0distribution. The solid black lines in (b–e) correspond to theoreticalΓ/Γ0distributions when considering isotropic dipole orientations for the dye molecules and fixed emitter–particle distances of 8 nm for the 50-bp DNA spacer (b,d) and 6 nm for the 30-bp DNA spacer (c,e). These distributions are corrected for the angle-dependent antenna efficiency. The dashed black lines in (b–e) are theoreticalΓ/Γ0distributions forθ=π/4 and Gaussian distributions ofdcentred at 6.5 nm and 8.25 nm for the 30 bp and 50 bp linkers, respectively. The s.d.'s ofdare ±0.5 nm for single particles (b,c) and ±1 nm for dimers (d,e). Figure 2 depicts the distributions of measured normalized decay rate enhancements Γ / Γ 0 , with Γ 0 the average decay rate of isolated ATTO647N molecules. This graph clearly demonstrates the drastically different behaviour of the five samples: not only does changing the emitter–particle distance in the nanometre range (10 bp) shift the rate enhancement distribution for single particles and dimers, but SMs in dimers consistently feature three times larger Γ / Γ 0 than in the vicinity of one AuNP. Furthermore, Fig. 2e for 30 bp dimers shows that rate enhancements close to two orders of magnitude are reproducibly observed. As organic molecules typically feature lifetimes in the nanosecond range, this corresponds to the maximum rate enhancements that can be unambiguously estimated using time-correlated single photon counting (~10 ps lifetimes) [10] . By shortening the DNA spacer or choosing a molecule emitting at the longitudinal dimer resonance (~550 nm in these experimental conditions) [14] , it would be possible to synthesize, but not to analyse, nanoantennas with three orders of magnitude decay rate enhancements. Figure 2: Distributions of decay rate enhancements Γ / Γ 0 . Isolated ATTO647N molecules ( a ), single AuNPs with 50 bp ( b ) and 30 bp ( c ) DNA spacers, and 50 bp ( d ) and 30 bp ( e ) dimers. Experimental bar widths are Δ Γ / Γ =Δ τ / τ =0.12. The solid black line in ( a ) is a Gaussian fit of the experimental Γ 0 / Γ 0 distribution. The solid black lines in ( b – e ) correspond to theoretical Γ / Γ 0 distributions when considering isotropic dipole orientations for the dye molecules and fixed emitter–particle distances of 8 nm for the 50-bp DNA spacer ( b , d ) and 6 nm for the 30-bp DNA spacer ( c , e ). These distributions are corrected for the angle-dependent antenna efficiency. The dashed black lines in ( b – e ) are theoretical Γ / Γ 0 distributions for θ = π /4 and Gaussian distributions of d centred at 6.5 nm and 8.25 nm for the 30 bp and 50 bp linkers, respectively. The s.d. 's of d are ±0.5 nm for single particles ( b , c ) and ±1 nm for dimers ( d , e ). Full size image Mie theory calculations To verify that the measured distributions correspond to the target antenna geometries, we computed Γ / Γ 0 using generalized Mie theory (GMT). GMT provides an analytical solution of Maxwell's equations for groupings of spheres in homogeneous dielectric environments, which is solved numerically up to a given multipolar order [24] (the bulk dielectric constant of gold [25] is used for the nanoparticles). Two parameters strongly modify the coupling efficiency between the metallic antenna and the fluorescent molecule, and can justify the wide Γ / Γ 0 distributions obtained in Fig. 2 : the angle between the SM transition dipole and the DNA strand, and the distance, d , between the molecule and the particle surface. The relative strength of quenching and radiative decay in Γ / Γ 0 is given by the ratio between radiated and total dissipated power when the antenna is driven by a classical electric dipole [26] . This ratio, η = Γ R / Γ , is called the antenna efficiency [2] , with Γ R / Γ 0 the radiative decay rate enhancement. When θ =0, the dye molecule is longitudinally coupled to the AuNPs and, for dimers with emitter–particle distances in the 5–10 nm range, the rate enhancement is maximum with optimum antenna efficiency (23%< η <42% estimated in GMT). When θ = π /2, the coupling is transverse and the dimers exhibit a dark mode (0.02%< η <2.4%) with minimum Γ / Γ 0 . For single particles, η becomes non-negligible in transverse coupling (0.5%< η <18%) but longitudinal coupling provides less far-field emission than in a dimer (14%< η <40%). To take into account that SMs coupled to dark modes cannot be observed in the far field, we compute theoretical Γ / Γ 0 distributions by multiplying an isotropic orientation distribution, sinθ, with the angle-dependent antenna efficiency, η ( θ ), before normalization. By estimating Γ / Γ 0 and Γ R / Γ 0 for different values of θ using GMT, we observe that both quantities feature a cos 2 θ dependence corresponding to dipole–dipole coupling (see Fig. 3a and b ) and can be expressed as a function of Γ / Γ 0 for a given molecule–particle distance d as shown in Fig. 3c and d . The solid black line in Fig. 2a is a Gaussian fit of the decay rate distribution Γ 0 / Γ 0 of isolated SMs. The solid black lines in Fig. 2b through Fig. 2e correspond to an isotropic angle distribution multiplied by η ( Γ / Γ 0 ) and convoluted by the Γ 0 / Γ 0 Gaussian distribution. The interparticle distance is the only free parameter and is set, respectively, at 12 nm ( Fig. 2c and e ) and 16 nm ( Fig. 2b and d ) for the 30 bp and 50 bp spacers, in good agreement with experimental gap lengths estimated in cryo-EM [14] . 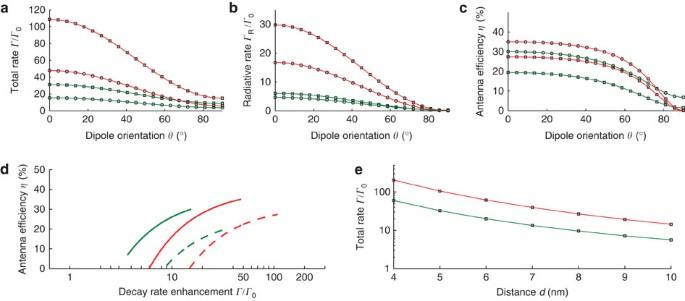Figure 3: Theoretical decay rates and antenna efficiencies. Evolution of the total (a) and radiative (b) decay rates, as well as the antenna efficiency (c), as a function of the emission dipole orientation,θ, for a fixed emitter–particle distance,d, of single emitters in the vicinity of a single 36 nm AuNP (green solid lines) and in the centre of a AuNP dimer (red solid lines).d=6 nm for the open squares and 8 nm for the open circles. The markers correspond to Mie theory calculations and the solid lines to a A+Bcos2(θ) fit of the decay rates. (d) Evolution of the antenna efficiencyη=ΓR/Γas a function ofΓfor 36 nm AuNPs (green lines) and dimers (red lines), obtained by combiningFig. 3a,c. The dashed lines correspond tod=6 nm and the solid lines tod=8 nm. (e) Evolution of the total decay rate for a single emitting dipole in the vicinity of a single 36 nm diameter AuNP (green solid line) or in the centre of a AuNP dimer (red solid line) forθ=π/4, as a function of the distance,d, between the emitter and the AuNP surface. The markers correspond to Mie theory calculations. Figure 3: Theoretical decay rates and antenna efficiencies. Evolution of the total ( a ) and radiative ( b ) decay rates, as well as the antenna efficiency ( c ), as a function of the emission dipole orientation, θ , for a fixed emitter–particle distance, d , of single emitters in the vicinity of a single 36 nm AuNP (green solid lines) and in the centre of a AuNP dimer (red solid lines). d =6 nm for the open squares and 8 nm for the open circles. The markers correspond to Mie theory calculations and the solid lines to a A+Bcos 2 (θ) fit of the decay rates. ( d ) Evolution of the antenna efficiency η = Γ R / Γ as a function of Γ for 36 nm AuNPs (green lines) and dimers (red lines), obtained by combining Fig. 3a,c . The dashed lines correspond to d =6 nm and the solid lines to d =8 nm. ( e ) Evolution of the total decay rate for a single emitting dipole in the vicinity of a single 36 nm diameter AuNP (green solid line) or in the centre of a AuNP dimer (red solid line) for θ = π /4, as a function of the distance, d , between the emitter and the AuNP surface. The markers correspond to Mie theory calculations. Full size image Small variations of the emitter–particle distance, d , can also induce a broad distribution of the Γ / Γ 0 enhancement values for a given transition dipole orientation. As mentioned earlier, cationic dyes tend to bind to DNA, hindering their rotational degrees of freedom [23] . In practice, large dye molecules typically interact with the DNA grooves, favouring a π /4 molecular orientation [27] . For θ = π /4, Γ / Γ 0 decreases nearly exponentially with d in the 4–10 nm range for both dimers and single gold particles (see Fig. 3e ). Therefore, a Gaussian distribution of d will correspond to a nearly log-normal distribution of Γ / Γ 0 . The dashed black lines in Fig. 2 correspond to a ±1 nm s.d. of d for the 50 bp and 30 bp dimers and a ±0.5 nm s.d. of d for the single particles with θ = π /4 (after convolution with the Gaussian Γ 0 / Γ 0 distribution). The centres of the Gaussian distributions are d =6.5 nm for the 30 bp spacer and 8.25 nm for the 50 bp spacer, respectively, in good agreement with cryo-EM data [14] . The factor of 2 between the s.d. 's of d for single particles and dimers is justified by the number of thiol-based flexible covalent links between the gold particles and the DNA double strand. The excellent correspondence between the measured Γ / Γ 0 distributions and the two theoretical ones indicates that the emitter–particle distance is effectively tuned by 2 nm when modifying the length of the DNA spacer, a scale unreachable with top–down lithography. Furthermore, the two theoretical distributions are extreme cases: fixed distance and isotropic orientation distribution for the solid lines, and fixed angle and ±0.5–1 nm s.d. 's of d for the dashed lines. Other experimental factors such as the particle size and shape distributions can further widen the theoretical distributions by a few tens of percents. In practice, our experiments probably correspond to an intermediate system with a limited distribution of molecular orientations and distance s.d. 's smaller than ±1 nm in dimers, further demonstrating the excellent position control offered by DNA templates. The theoretical efficiencies estimated in Mie calculations, for an emission wavelength of 670 nm, indicate that at a given emitter–particle distance, dimers allow three times larger rate enhancements with higher η (see Fig. 3d ). In particular, to match the Γ / Γ 0 enhancement of a 30 bp dimer in longitudinal coupling with a single particle, the molecule should be <4 nm away from the gold surface with η =8% compared with η =27% in the dimer. Theoretical efficiencies are, however, smaller than the initial ATTO647N quantum yield (65%) and will result in quenching. 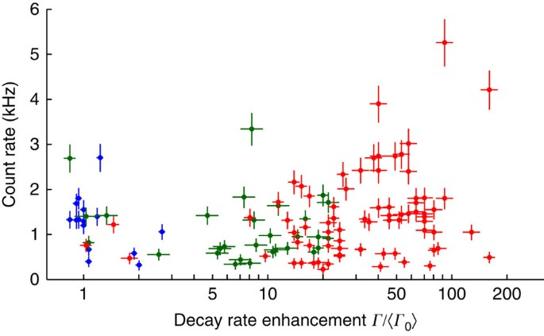Figure 4: Fluorescence count rates. Distribution of SM count rates versusΓ/Γ0for isolated molecules (blue data points), single AuNPs with 30 bp and 50 bp spacers (green points), and 30 bp and 50 bp dimers (red points). This plot corresponds to all measurements featuring a clear bleaching step. The horizontal error bars are the monoexponential fitting uncertainties Δτ/τ=ΔΓ/Γthat vary between 0.05 and 0.3. Vertical bars correspond to a 20% error, typically observed in the time traces. Figure 4 provides the measured count rates of SMs before bleaching versus Γ / Γ 0 . The wide data dispersion is due to different out-of-plane orientations of the dye molecules that forbid a direct estimation of the effective quantum yields. However, Fig. 4 already demonstrates that SMs coupled to AuNP dimers can feature a two-order of magnitude Γ / Γ 0 enhancement and an increased photon flux. Figure 4: Fluorescence count rates. Distribution of SM count rates versus Γ / Γ 0 for isolated molecules (blue data points), single AuNPs with 30 bp and 50 bp spacers (green points), and 30 bp and 50 bp dimers (red points). This plot corresponds to all measurements featuring a clear bleaching step. The horizontal error bars are the monoexponential fitting uncertainties Δ τ / τ =Δ Γ / Γ that vary between 0.05 and 0.3. Vertical bars correspond to a 20% error, typically observed in the time traces. Full size image The highest count rates were consistently observed in the 30-bp dimer sample while the lowest count rates were measured when the dye molecules are linked to a single particle with a 30 bp spacer. The lower effective quantum yield of ATTO647N molecules in the vicinity of nanoantennas is thus compensated by excitation enhancement in the case of dimers but not with single 36 nm diameter particles. Therefore, while single particles induce stronger fluorescence signal quenching as the distance decreases [13] , dimers exhibit higher count rates for shorter spacings. Dye molecules with low initial quantum yield would allow larger count rate enhancements [10] , [28] but their initial shorter lifetimes would forbid the measurement of high Γ / Γ 0 enhancements as given in Fig. 2 . In practice, experimental estimation of the antenna efficiencies would require knowing precisely the orientation of the DNA linkers in the microchamber or averaged fluorescence correlation spectroscopy measurements [28] . Compared with large top–down-fabricated gold antennas [10] , colloidal AuNPs induce a weak background signal in fluorescence time traces. This allows us to measure photon antibunching [29] in SM-driven DNA-templated dimers as shown on Fig. 5 in comparison with isolated ATTO647N molecules. The observed peak narrowing in the emission statistics of the nanoantenna demonstrates increased temporal coherence from a quantized emitter. 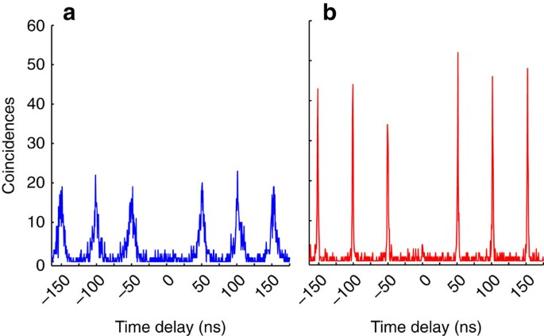Figure 5: Photon antibunching measurements. Typical photon emission statistics of (a) an isolated ATTO647N and (b) a 30 bp dimer (average 5–8-kHz count rate on both APDs). Figure 5: Photon antibunching measurements. Typical photon emission statistics of ( a ) an isolated ATTO647N and ( b ) a 30 bp dimer (average 5–8-kHz count rate on both APDs). Full size image In this work, ATTO647N molecules were introduced in the vicinity of single gold particles or in the centre of AuNP dimers using one DNA double strand. Excellent agreement between theoretical calculations and experimental data demonstrates a nanometre control over the emitter position in the centre of the dimers. Larger decay rate enhancements and fluorescence count rates with better antenna efficiencies are achieved in dimers compared with single AuNPs. In practice, dye molecule-driven dimers are obtained in easily processable, high-purity suspensions, and exhibit accelerated single photon emission. These self-assembled nanoantennas are ideal model systems to investigate experimentally how bright and dark electromagnetic environments not only enhance [10] or shape [11] spontaneous emission but also mediate long-distance energy transfer and photochemical processes for efficient light harvesting and energy conversion [30] . Sample fabrication Citrate-coated 36-nm-diameter gold nanoparticles (AuNPs) were purchased from BBInternational (UK), and PAGE-purified trithiolated DNA sequences with a single ATTO647N molecule in the centre (respectively, attached to amino-modified C and A bases) were obtained from Fidelity Systems, Inc (USA). Nanoparticle surface ligand exchanges, DNA hybridization and electrophoretic purifications are performed using published procedures [14] . Fluorescence measurements Biotin-functionalized single particles and dimers are grafted on the surface of home-made Neutravidin-coated microfluidic chambers using methods described elsewhere [14] . An oxygen scavenger (10 mM protocatechuic acid and 200 nM protocatechuate-3,4,dioxygenase) [20] and reducing and oxidizing agents (1 mM ascorbic acid and methyl viologen) [21] , [22] are added in the final 50 mM NaCl/10 mM Tris buffer (pH=8) before sealing the microchamber with hot wax. The sample is illuminated in an inverted microscope (Olympus IX71) using a 1.3 NA objective with an unpolarized supercontinuum laser (SC450-pp, Fianium), spectrally filtered around 635 nm, which delivers 50-ps pulses at a 10-MHz repetition rate. The fluorescence signal is imaged on an EMCCD camera (Ixon, Andor) or focused on an APD (MPD-5CTC) after spatial filtering through a 100-μm confocal pinhole. Time-correlated single photon counting (Hydraharp 400, Picoquant) is used to estimate the fluorescence lifetime of SMs. Antibunching measurements are performed in a Hanbury, Brown and Twiss architecture with a second identical APD, separated from the first by a 50/50 beamsplitter. In that case, the excitation intensity is of the order of 1 kW cm −2 with a 20-MHz repetition rate. Theoretical calculations Calculations are performed using an in-house GMT code [24] . The emission wavelength is set at 670 nm and the particle diameter at 36 nm. The refractive index of the surrounding medium is set at 1.4 for comparison with experiments performed at inhomogeneous glass–water interfaces [13] , [14] while the dielectric constant of gold is tabulated from published data [25] . Calculations are performed with a multipole order n =30. How to cite this article: Busson, M.P. et al . Accelerated single photon emission from dye molecule-driven nanoantennas assembled on DNA. Nat. Commun. 3:962 doi: 10.1038/ncomms1964 (2012).